Baiji genomes reveal low genetic variability and new insights into secondary aquatic adaptations The baiji, or Yangtze River dolphin ( Lipotes vexillifer ), is a flagship species for the conservation of aquatic animals and ecosystems in the Yangtze River of China; however, this species has now been recognized as functionally extinct. Here we report a high-quality draft genome and three re-sequenced genomes of L. vexillifer using Illumina short-read sequencing technology. Comparative genomic analyses reveal that cetaceans have a slow molecular clock and molecular adaptations to their aquatic lifestyle. We also find a significantly lower number of heterozygous single nucleotide polymorphisms in the baiji compared to all other mammalian genomes reported thus far. A reconstruction of the demographic history of the baiji indicates that a bottleneck occurred near the end of the last deglaciation, a time coinciding with a rapid decrease in temperature and the rise of eustatic sea level. The baiji, or Yangtze River dolphin ( Lipotes vexillifer ), is endemic to the middle and lower reaches of the Yangtze River of China. Nicknamed ‘Goddess of the Yangtze’ or ‘panda in water’, the baiji has become one of the most famous species in aquatic conservation. Unfortunately, this species has experienced a catastrophic population collapse in recent decades due largely to various extreme anthropogenic pressures [1] . Although great efforts have been made to conserve the baiji, the most recent internationally organized survey, which was conducted in late 2006, failed to identify any living individuals. This led the survey organizers to declare it functionally extinct [2] . In addition to being a symbol of conservation, as a fully sequenced genome from the order Cetacea, the baiji genome is also unique in an evolutionary and phylogenetic context. Particularly, cetaceans (whales, dolphins, and porpoises), which represent 4% of the mammalian diversity, are adapted to a permanent aquatic life and exhibit with distinctive and highly specialized characteristics including (but not limited to) loss of external hind limbs, echolocation, and changes in respiratory and cardiovascular anatomy and physiology, thereby diverging from the other mammalian orders [3] , [4] . Furthermore, paleontological, morphological, and molecular evidence has suggested that cetaceans are nested within Artiodactyla and became secondarily aquatic more than 50 million years ago, accompanied by a long ‘ghost’ lineage, masking the origin of this group of mammals [5] . Thus, adequate genomic information from this group is critical for understanding the evolutionary history and myriad of adaptations in cetaceans. Here, using a whole-genome shotgun strategy and Illumina Hiseq2000, we report a draft genome sequence with ~114x coverage for a male baiji. Comparative genomic analyses provide insight into the evolutionary adaptations of cetaceans and the genetic basis underlying the recent demographic decline of the baiji. In addition, the genome provides valuable resources for further research on the biology and conservation of mammals and cetaceans in particular. Genome sequencing and assembly We applied a whole-genome shotgun strategy to sequence the genome of a single non-breeding male baiji. After filtering low-quality and duplicated reads, 320.87 Gb (approximately114.6-fold coverage) of clean data were retained for assembly ( Supplementary Table S1 ). The genome size was estimated to be 2.8 Gb based on the frequency distribution of 17-base oligonucleotides (17-mer) in the usable sequencing reads and the sequencing depth [6] ( Supplementary Fig. S1 and Supplementary Table S2 ), which is comparable to cow (2.87 Gb) and horse (2.7 Gb). The final genome assembly was 2.53 Gb (contigs), with contig and scaffold N50, values of 30 kb and 2.26 Mb, respectively ( Supplementary Table S3 ). Approximately 90% of the total sequence was contained in the 1,295 longest scaffolds (>345 kb), with the largest scaffold spanning 11.54 Mb. The assembly metrics of the baiji genome were comparable to those of other animal genomes generated using next-generation sequencing technology (NGS) [7] ( Supplementary Table S3 ). The peak sequencing depth was 102-fold and 99% of the genome assembly was more than 50-fold ( Supplementary Fig. S2 ). In general, the average GC content of the baiji was similar to that of other mammals, and all genomic regions with GC contents between 30% and 70% had more than 50-fold coverage ( Supplementary Figs S2 and S3 ). To assess the large-scale and local assembly accuracy of the scaffolds, 17 fosmid library clones were independently sequenced and assembled using shotgun sequencing technology. Most of the fosmid clones were best aligned to only one scaffold, and no obvious misassembly was observed ( Supplementary Table S4 and Supplementary Fig. S4 ). Similar to other well-annotated mammalian genomes, approximately 43% of the baiji genome comprised transposon-derived repeats, and the predicted baiji gene set contained 22,168 genes ( Fig. 1a ; Supplementary Tables S5–S8 ). Based on homology approaches, more than 98% of baiji genes showed similarity with functionally known genes of five frequently used databases ( Supplementary Table S9 ). We identified 55,639 recent segmental duplications (SDs) (>1 kb in length,>90% identity) with a total length of 51.3 Mb (~2%) in the baiji genome, which is less than what was observed in human and mouse but more than in giant panda ( Supplementary Table S10 and Supplementary Figs S5 and S6 ). In the baiji genome, genes in SDs were significantly enriched in the gene ontology (GO) terms ‘cytoskeleton’ (GO:0005856, P =6.68 × 10 −15 , hypergeometric test), ‘GTPase activity’ (GO:0003924, P =2.69 × 10 −9 , hypergeometric test), and ‘microtubule-based process’ (GO:0007017, P =4.13 × 10 −9 , hypergeometric test). 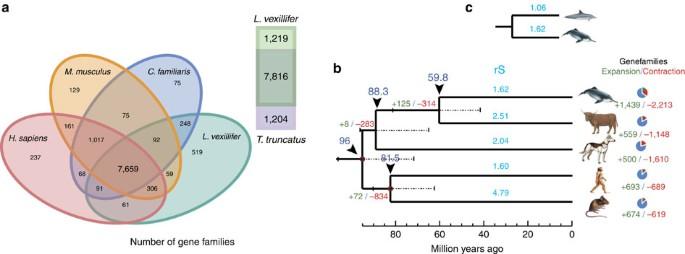Figure 1: Comparison of gene families and the phylogenetic tree. (a) Venn diagram showing unique and overlapping gene families in the baiji, common bottlenose dolphin, dog, human, and mouse. (bandc) Phylogenetic tree and divergence times estimated for the baiji and other mammals. Numbers associated with each terminal branch in light blue are mean rates of synonymous substitution values (rS). Numbers associated with each branch designate the number of gene families that have expanded (green) and contracted (red) since the split from the common ancestor. Triangle arrows and the numbers under them denote the most recent common ancestor (TMCRA), and the scale units are million years ago. The standard error range for each age is represented by the dashed line. The red solid circles on the branch nodes denote the node as an ‘age constraint’ used in the estimation of the time of divergence. Figure 1: Comparison of gene families and the phylogenetic tree. ( a ) Venn diagram showing unique and overlapping gene families in the baiji, common bottlenose dolphin, dog, human, and mouse. ( b and c ) Phylogenetic tree and divergence times estimated for the baiji and other mammals. Numbers associated with each terminal branch in light blue are mean rates of synonymous substitution values (rS). Numbers associated with each branch designate the number of gene families that have expanded (green) and contracted (red) since the split from the common ancestor. Triangle arrows and the numbers under them denote the most recent common ancestor (TMCRA), and the scale units are million years ago. The standard error range for each age is represented by the dashed line. The red solid circles on the branch nodes denote the node as an ‘age constraint’ used in the estimation of the time of divergence. Full size image Substitution rate and turnover of gene families The rates of molecular evolution vary in different lineages and can be inferred by estimating the rate at which neutral substitutions accumulate in protein-coding genes [8] . Previous studies have suggested that the point mutation rate has decreased in apes, especially in humans (the ‘hominid slowdown’) [9] , [10] , and studies have indicated that whales have a slow molecular clock [11] . The baiji genome enables an estimation of the rate of neutral substitutions in Cetacea, and Odontoceti in particular, because single copy genes and fourfold degenerate sites were sampled. All terminal lineages have similar mean dN/dS (the ratio of the rate of non-synonymous substitutions to the rate of synonymous substitutions) values except for the baiji ( Supplementary Table S11 and Supplementary Fig. S7 ). The high value of dN/dS in the baiji arose from a low dS rather than a high dN, indicating a comparatively low substitution rate and slower molecular clock in cetaceans. The mean rates of synonymous substitution (rS) along the cetacean lineage (baiji and the bottlenose dolphin) are the slowest among the seven mammalian branches measured ( Fig. 1b and Supplementary Table S12 ). Additionally, the rates of synonymous substitution in cetaceans, especially in the baiji, were comparable to that of the human lineage [12] . The absolute rates for each species also revealed that substitution rates in cetaceans (1.22 × 10 −9 substitutions per site per year for baiji and 0.84 × 10 −9 substitutions per site per year for the common bottlenose dolphin) were lower than those for the other species in our comparative set and lower than the average mammalian mutation rate [13] . The mechanistic basis for the mutation rate variation in mammalian genomes is mostly unclear [14] , and previous studies suggested that lineage-specific rate variation might be correlated with some species-specific biological features, particularly in mammals [15] . The single variable regressions conducted with the present dataset support the notion that species with greater mass or longer generation times have lower rates of substitution (generation time, rS: slope=−0.71, r 2 =0.82, P =0.003; body weight, rS: slope=−0.25, r 2 =0.59, P =0.0274) ( Supplementary Table S12 ). We determined the expansion and contraction of gene ortholog clusters, which showed that the baiji has undergone twice the amount of variation of in gene families compared with the other mammals examined ( Fig. 1b ). Among the gene families that underwent the most significant turnover in the baiji, genes involved in oxidoreductase activity (GO:0016491, P =5.54 × 10 −54 , hypergeometric test), ferric iron binding (GO:0008199, P =1.35 × 10 −43 , hypergeometric test), metabolic processes (GO:0008152, P =2.04 × 10 −10 , hypergeometric test), and ATPase activity (GO:0016887, P =2.04 × 10 −10 , hypergeometric test) were found to have expanded significantly, whereas genes involved in olfactory receptor activity (GO:0004984, P =2.914 × 10 −85 , hypergeometric test) decreased most significantly. Both changes may be correlated with the basic physiological activities required for underwater living, such as oxygen carrying and sensing. Pseudogenes have also been identified, which were mainly involved in binding (GO:0005488, 63.9%), cell part (GO:0044464, 43.9%), metabolic process (GO:0008152, 41.6%), and catalytic activity (GO:0003824, 33.3%) ( Supplementary Table S13 and Supplementary Fig. S8 ). Many genes associated with pigmentation (GO:0043473, 15.3%) were pseudogenes, which might relate to the overall dull color and simplistic skin pigmentation pattern in the baiji. PSGs and molecular adaptation in cetaceans Investigating positively selected genes (PSGs) in the baiji genome can provide insights into the secondary aquatic adaptations of this unique group of mammals. Of the 10,423 1:1 orthologues from the six species shown in Fig. 1b,c , 423 PSGs were found in the baiji lineage and 24 PSGs were found in the common branch to the baiji and dolphin ( Supplementary Table S14 ) using the branch site-mode [16] under a conservative 1% false-discovery-rate criterion with a Bonferroni correction of less than 0.01. The relatively large number of PSGs in the baiji could have resulted from a generally higher mean dN/dS along the cetacean lineage ( Supplementary Fig. S7 ). GO classification of the baiji PSGs reflects gene enrichment in protein binding (GO:0005515, P =0.00017, hypergeometric test), cellular process (GO:0009987, P =0.022, hypergeometric test), and intracellular signal transduction (GO:0035556, P =0.036, hypergeometric test). It should be noted that PSGs in the baiji lineage were also involved in DNA repair (GO:0006281) and response to DNA damage stimulus (GO:0006974), which have not been noted in previous analyses of mammals [17] or dolphin [18] , [19] . Pathways related to DNA repair and damage are known to have a major impact on the development of the brain and have been implicated in diseases such as microcephaly [20] , [21] , whereas the evolution of DNA damage pathways might also have contributed to the slowdown of the substitution rate [22] , which was observed in cetaceans. In addition to positive selection, the aquatic adaptations of cetaceans could be driven by other functional changes. For example, river dolphins, such as the baiji, have convergently reduced the size of their eyes and the acuity of their vision, likely in response to poor visibility in fluvial and estuarine environments [23] . Upon examining 209 genes related to vision in humans (GO:0007601: visual perception) in the baiji genome, we identified four genes ( OPN1SW , OPN3 , ARR3 , and PDZD7 ) that may have lost their function due to a frameshift mutation or premature stop codons ( Supplementary Table S15 ). Of the three essential opsins in mammals, baiji possess the inactivated short wavelength-sensitive opsin (SWS1), functional rod opsin (RH1), and long wavelength-sensitive opsin (LWS), similar to most of the toothed whales [24] , [25] . Odontocete cetaceans have also evolved a complex system of echolocation that involves the production and perception of high-frequency sound under water [4] . The independent origin of echolocation in toothed whales and echolocating bats is a classic model of convergent evolution [26] , [27] . Previous genetic studies have documented parallel sequence evolution and positive selection in five genes in bats and dolphins ( SLC26A5 , Cdh23 , Pcdh15 , TMC1 , and DFNB59 ) [26] , [27] , [28] , [29] . When combined with the assembly of the little brown bat ( Myotis lucifugus ), 74 1:1 orthologs of candidate genes associated with hearing and vocalization were identified and examined in Myotis and the five species in Fig. 1b . To identify genes exhibiting convergent evolution in the baiji and Myotis lineages, the dN/dS of branches leading to echolocating mammals (ω2) were estimated and compared to those of all other branches (ω1) as well as to the average ω across the tree (ω0). Seven genes (including SLC26A5 and TMC1 ) were found to have evolved under significant accelerated evolution ( Table 1 ), and 17 genes contained parallel amino acid changes in echolocating mammals ( Supplementary Table S16 ). Table 1 Tests of accelerated and parallel evolution of genes associated with hearing and vocalization in baiji and the little brown bat. Full size table A previous study revealed that genes encoding sweet, umami, and bitter taste receptors were nonfunctional in the bottlenose dolphin [30] . We confirmed these results, and further, we discovered that all taste receptor genes in the baiji and dolphin are pseudogenes, with the exception of the salt receptor ENaC, a hetero-oligomeric complex comprising by three homologous subunits ( SCNN1A , SCNN1B , and SCNN1G ) ( Supplementary Tables S17 and S18 ). Secondarily aquatic amniotes also have reduced olfactory capacity; 248 olfactory receptor (OR) genes can be identified in the baiji genome ( Supplementary Table S19 ), which is less than that in many other mammals [31] , [32] . As in other cetaceans, nearly half of the OR genes (49%), as well as TRPC2 , are potentially nonfunctional due to frameshifts and/or inserted stop codons. Our results revealed that OR gene family groups 1/3/7 (25%) and 2/13 (23%) had the highest proportion of functional ORs in the baiji, suggesting that these genes might assume other functions in addition to olfaction [31] . The massive loss of ORs in the baiji genome is consistent with the complete loss of the olfactory bulb or olfactory tract in odontocetes [33] , [34] . Heterozygosity rate and demographic history The baiji genome provides us the opportunity to investigate what role, if any, the genome played in the functional extinction of this organism. We used the assembled baiji genome sequence as a reference and realigned all usable sequencing reads from all four sequenced individuals. A total of 825,504 and 672,755 heterozygous single nucleotide polymorphisms (SNPs) were identified with the most relaxed and stringent filters, respectively. Of the 683 genes with SNPs, genes involved in protein complex (GO:0043234, P =0.006, hypergeometric test), plasma membrane (GO:0005886, P =0.02, hypergeometric test), protein binding (GO:0005515, P =4.66 × 10 −5 , hypergeometric test), and cell adhesion (GO:0007155, P =0.01, hypergeometric test) were significantly enriched. 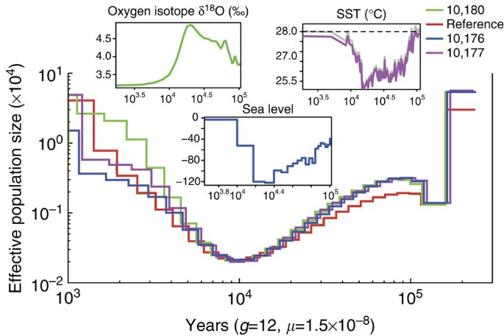Figure 2: Demographic histories of the baiji reconstructed using the PSMC model. Smoothed curves on the top represent global climate39, sea surface temperature (SST) of South China Sea40, and global sea-level fluctuations41. Horizontal dashed line marks present SST for modern times. The age units for all graphs are years. The estimated mean heterozygosity rate of the baiji genomes was 1.21 × 10 −4 ( Table 2 and Supplementary Table S20 ), which is approximately 11 times lower than the rate estimated for the panda genome (1.32 × 10 −3 ) [35] , [36] , another critically endangered animal, and approximately 6 times lower than that of naked mole rat (0.7 × 10 −3 ) which was recognized as an inbreeding species [37] . The heterozygosity rate in the X chromosome was about 73% that of the autosomes and Y chromosome, and the transition/transversion ratio was 1.40 ( Table 2 ). To our knowledge, the baiji has the lowest SNP frequency of all other individual mammalian genomes reported thus far. This low frequency could be related to the relatively low rate of molecular evolution in cetaceans; however, considering that the decrease in the rate of molecular evolution in the baiji was not as great as the decrease in the heterozygosity rate, it is likely that much of the low genetic diversity observed was caused by the precipitous decline in the total baiji population in recent decades and the associated inbreeding. Table 2 Statistics of identified heterozygous SNPs in baiji genomes. Full size table A reconstruction of the population demography of the baiji uncovered a historical bottleneck, which may have contributed to its low level of genetic variability. The pairwise sequentially Markovian coalescent (PSMC) model [38] was used to examine the changes in the local density of heterozygotes across the baiji genome and to reconstruct its demographic history. Our analyses uncovered distinct demographic trends from 100,000 to 1,000 years ago ( Fig. 2 and Supplementary Fig. S9 ); the baiji experienced a consistent and unidirectional contraction of its population with the smallest effective population size (bottleneck) ~10 thousand years ago (KYA ). The population then expanded to reach its greatest size ~1 KYA. Overall, our reconstructed demographic history correlates well with global climate [39] and the Pleistocene and Holocene temperature record of the South China Sea with one major exception [40] : the nadir of population size postdates the nadir in temperature by approximately 10 KYA. One possible explanation for this inconsistency is that the population size of the baiji was influenced by temperature and rates of sea level rise [41] . The smallest population coincides with the last deglaciation and the most rapid rises in eustatic sea level over the last 100 KYA (approximately 1–1.5 cm/yr). The rapid rise in sea level would have drowned the Yangtze River valley and led to a dramatic reduction in available freshwater habitats. Once the rate of rise slowed, the now submerged valley would have infilled [42] , and the resulting decrease in the river gradient would have led to a more complex river system (i.e., meanders, gradients) and new habitats for recovering baiji populations. Regardless of the exact cause(s) of the historical bottleneck, the constant population growth after 10 KYA indicates that the recent declines and eventual functional extinction of the baiji are not a direct consequence of this historical bottleneck but instead were caused by extreme human impacts to the Yangtze River in recent decades [1] . Figure 2: Demographic histories of the baiji reconstructed using the PSMC model. Smoothed curves on the top represent global climate [39] , sea surface temperature (SST) of South China Sea [40] , and global sea-level fluctuations [41] . Horizontal dashed line marks present SST for modern times. The age units for all graphs are years. Full size image We found a generally slow substitution rate in cetaceans through genome sequencing of the Yangtze River dolphin and comparative analyses with other mammalian genomes. New insights into potential molecular adaptations to secondary aquatic life were outlined, such as a decrease in olfactory and taste receptor genes, changes in vision and hearing genes, and positive selection on genes related to expansion of the brain. Notably, baiji genomes have the lowest density of SNPs among the available mammal genomes, which is consistent with the small and rapidly declining population size of this organism. The reconstructed demographic history over the last 100 KYA featured a continual population contraction through the last glacial maximum, a serious bottleneck during the last deglaciation, and sustained and rapid population growth after the eustatic sea level approached the current levels. The close correlation between population trends, regional temperatures, and eustatic sea level suggests a dominant role for global and local climate changes in shaping the baiji’s ancient population demography. Future genetic sequencing from additional individuals would allow for further reconstruction of the demographic history of the baiji, allow us to test our hypothesis regarding the correlation between baiji population dynamics and global climate fluctuations, and uncover the role of genetic factors in the functional extinction of this organism. Baiji samples An adult male baiji that has been stored at Nanjing Normal University at −20 °C since 1985 was chosen for de novo sequencing. One male and two female animals were used for resequencing. Genomic DNA was extracted from abdominal muscle and the quality and quantity of DNA obtained was sufficient for whole-genome sequencing. Genome sequencing and assembly Libraries for genomic DNA sequencing were constructed according to the Illumina standard protocol. In total, 22 standard libraries (insert size=180 bp to 20 kb) and one PCR-free library (insert size=350 bp) were constructed and sequenced using an Illumina Hiseq2000. Finally, 503.87 Gb of raw data were generated, and after filtering, 320.8 Gb of data remained for de novo assembly. Whole-genome assembly was performed using SOAP denovo [43] , and Gapcloser (version1.12, http://soap.genomics.org.cn/soapdenovo.html ) was used to fill gap (N) regions. Additionally, 17 fosmid clones were sequenced using Sanger methods and used as reference data to determine genomic coverage. Genome annotation and evolution Interspersed repeats were characterized by homolog-based identification using RepeatMasker ( http://www.repeatmasker.org ) and the repeat database, Repbase [44] . Repeated proteins were identified using RepeatProteinMask, and de novo interspersed repeat annotation was performed using RepeatModeler ( http://www.repeatmasker.org/RepeatModeler.html . ). An additional round of RepeatMasker analysis was applied following de novo repeat identification. All repeats identified in this way were defined as total interspersed repeats. Tandem repeats were identified using Tandem Repeat Finder [45] . Protein sequences from cow, dog, horse, human, mouse, and dolphin were obtained and aligned against the baiji genome assembly using tblastn [46] . Loci with aligned proteins were extracted, and GeneWise [47] was used to predict the gene model. Augustus [48] , GENSCAN [49] , and GlimmerHMM [50] were used for de novo gene prediction. GLEAN [51] was applied to integrate the predicted genes and form the final gene set. To infer gene functions, we searched the final gene set against the protein databases KEGG [52] , SwissProt [53] , and TrEMBL [54] . InterProScan (Pfam, PRINTS, PROSITE, ProDom, and SMART databases) [55] was used to determine motifs and domains in the final gene set. Phylogenetic analyses and substitution rate The phylogenetic tree was constructed in MrBayes 3.1.2 (ref. 56 ) using single-copy orthologous genes ( Supplementary Methods ). The best-fit model was determined using MRMODELTEST 2.3 (ref. 57 ). Bayesian molecular dating was adopted to estimate the neutral evolutionary rate and species divergence time using MCMCTREE, implemented in PAML (v. 4.4b) [16] . Branch-specific evolutionary analyses of selection pressure were conducted on concatenated alignments using the free ratio model of the codeml package in PAML [16] . The absolute neutral substitution rate per year (nt/years) was estimated under both global [58] and local clock models, using baseml within PAML [16] . Positively selected genes and demographics The branch-site model [59] was used to detect positive selection along a target branch. We compared Model A1, in which sites may evolve either neutrally or under purifying selection, with Model A, which allows sites to be under positive selection. SOAPsnp (version 1.15) [60] , which uses a Bayesian statistical model, was used to call heterozygous SNPs in the baiji assembly. The recently developed PSMC model [38] was utilized to estimate demographic history using heterozygous sites across the genome. Accession Codes The whole genome sequences have been deposited at DDBJ/EMBL/GenBank nucleotide core database under the accession AUPI00000000 . The version described in this paper is version AUPI01000000 . How to cite this article: Zhou, X. et al . Baiji genomes reveal low genetic variability and new insights into secondary aquatic adaptations. Nat. Commun. 4:2708 doi: 10.1038/ncomms3708 (2013).